Genome analysis reveals insights into physiology and longevity of the Brandt’s batMyotis brandtii Bats account for one-fifth of mammalian species, are the only mammals with powered flight, and are among the few animals that echolocate. The insect-eating Brandt’s bat ( Myotis brandtii ) is the longest-lived bat species known to date (lifespan exceeds 40 years) and, at 4–8 g adult body weight, is the most extreme mammal with regard to disparity between body mass and longevity. Here we report sequencing and analysis of the Brandt’s bat genome and transcriptome, which suggest adaptations consistent with echolocation and hibernation, as well as altered metabolism, reproduction and visual function. Unique sequence changes in growth hormone and insulin-like growth factor 1 receptors are also observed. The data suggest that an altered growth hormone/insulin-like growth factor 1 axis, which may be common to other long-lived bat species, together with adaptations such as hibernation and low reproductive rate, contribute to the exceptional lifespan of the Brandt’s bat. Bats are among the most successful groups of animals. They account for ~20% of mammalian species, are the only mammals that have evolved powered flight, and are among the few animals that echolocate [1] . Bats are also among the smallest of mammals, but are unusually long-lived, thus challenging the observed positive correlation between body mass and maximum lifespan [2] . The Brandt’s bat ( Myotis brandtii ) holds the record with regard to lifespan among the bats. Its reported maximal lifespan of at least 41 years also makes it the most extreme mammal with regard to disparity between body mass and longevity [3] . These animals reside in temperate areas throughout Europe and Asia, resting during the day, feeding at night and hibernating during winter. As of yet, however, these highly specialized animals have escaped detailed genome characterization. In this study, we present a genome and transcriptome of the Brandt’s bat. Their analyses revealed adaptations that this exceptionally long-lived animal developed for echolocation, hibernation, reproduction and visual function. We identified unique sequence changes in the growth hormone (GH) receptor (GHR) and insulin-like growth factor 1 (IGF1) receptor (IGF1R), which appear to be common to other long-lived bat species and contribute to the small body size and long lifespan of the Brandt’s bat. Genome sequence assembly and annotation A whole-genome shotgun strategy was applied to sequence the genome of an adult male Brandt’s bat ( M. brandtii ) from the Obvalnaya cave in Russia ( Fig. 1 and Supplementary Fig. S1 ; Supplementary Note 1 ). We also sequenced liver, kidney and brain transcriptomes of hibernating and summer-active M. brandtii . 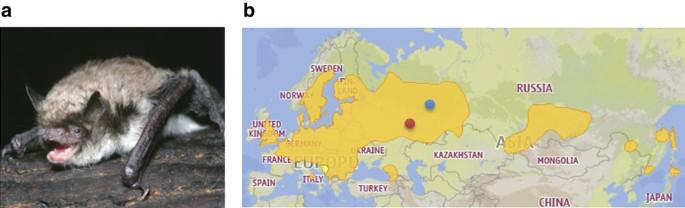Figure 1: Species map ofM. brandtii. (a)M. brandtii. (b) Occurrence ofM. brandtiiand areas of sample collection. Coloured dots indicate the location of sampled hibernating (December and April; shown in blue) and summer-active (June; shown in red) animals. Approximately 156 Gb (or 78 × ) genome data including 101 Gb (or 51 × ) short insert size reads were generated, resulting in a high-quality assembly with scaffold N50 of 3.1 Mb and contig N50 of 21 kb ( Table 1 , Supplementary Tables S1–S3 , Supplementary Figs S2,S3 ). The prevailing theory is that bats and birds have smaller genomes than other vertebrates due to metabolic constraints on cell size and, therefore, genome size [4] , [5] . Consistent with previous findings [6] , the M. brandtii genome size was smaller (~2 Gb) than other mammals ( Supplementary Fig. S2 ). Nucleotide diversity (per nucleotide heterozygosity) was estimated at 0.4%, higher than in another long-lived mammal, the naked mole rat [7] ( Supplementary Table S4 ). Known transposon-derived repeats accounted for 22% of the genome, which is lower than in related mammals and may contribute to the small size of the M. brandtii genome ( Supplementary Table S5 ). The predicted gene set included 22,256 protein-coding genes ( Supplementary Table S6 and Supplementary Fig. S4 ), of which 21,219 (95.3%) genes were transcribed (based on the RNA-seq data) and 20,744 (93.2%) genes could be functionally annotated by homology approaches ( Supplementary Table S7 ). Figure 1: Species map of M. brandtii . ( a ) M. brandtii . ( b ) Occurrence of M. brandtii and areas of sample collection. Coloured dots indicate the location of sampled hibernating (December and April; shown in blue) and summer-active (June; shown in red) animals. Full size image Table 1 Global statistics of the M. brandtii genome. Full size table Genome evolution The order of bats (Chiroptera) consists of Yangochiroptera (includes the Brandt’s bat and other echolocating bats) and Yinpterochiroptera (includes megabats, as well as some echolocating bat species), and belongs to the group of laurasiatherian mammals (together with Carnivora including dog and cat, Cetartiodactyla including cow and dolphin, Perissodactyla including horse, Eulipotyphla and Pholidota) 1 . To gain insight into the evolutionary relationships of bats, 2,654 single-copy orthologous genes were obtained from M. brandtii and eight related mammals and used to construct a phylogenetic tree ( Supplementary Fig. S5 ). High bootstrap evidence supported bats as the sister taxon of the horse ( Equus caballus ), although the remote estimated divergence date of ~81.7 million years ago is close to the time of mammalian radiation ( Fig. 2 ). This inference is also supported by comparing orthologous proteins ( Supplementary Fig. S6 and Supplementary Table S8 ) and by recent findings at the transcript level [8] , [9] . Interestingly, both M. brandtii and E. caballus are long-lived species, but differ dramatically in body size. Compared with the common ancestor of bats and horses, M. brandtii has 67 significantly expanded and 44 significantly contracted gene families ( Fig. 2 and Supplementary Fig. S7 ). Many expanded gene families in the Brandt’s bat are involved in the immune response, for example, IPR003599 immunoglobulin subtype and IPR003596 immunoglobulin V-set subgroup ( Supplementary Data 1 ), which is consistent with previous studies on bats in general. We found that many olfactory receptor gene families underwent contraction in the M. brandtii lineage ( Supplementary Data 2 ), which may reflect that M. brandtii depends primarily on echolocation and vision for sensory perception. Indeed, the olfactory system is aberrant in many bats, including the related M. lucifugus [10] , [11] . 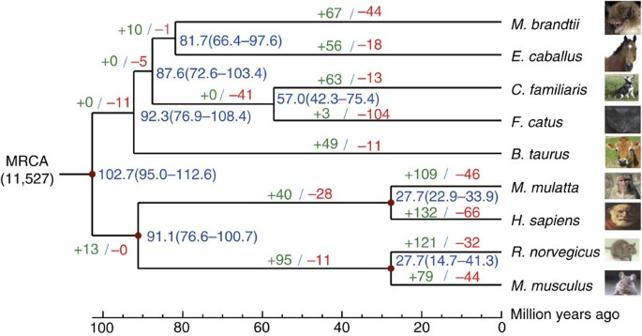Figure 2: Relationship ofM. brandtiito other mammals. Consensus phylogenetic tree shows the relationship among nine mammals based on 2,654 single-copy genes. The divergence times for all nodes were estimated based on the four red nodes with fossil records as calibration times and marked in each node with error range. Gene family expansion events are marked in green, and gene family contraction events in red. MRCA refers to the gene family number of the most recent common ancestor. Figure 2: Relationship of M. brandtii to other mammals. Consensus phylogenetic tree shows the relationship among nine mammals based on 2,654 single-copy genes. The divergence times for all nodes were estimated based on the four red nodes with fossil records as calibration times and marked in each node with error range. Gene family expansion events are marked in green, and gene family contraction events in red. MRCA refers to the gene family number of the most recent common ancestor. Full size image Analysis of syntenic regions identified 349 gained and 98 lost M. brandtii genes ( Supplementary Tables S9,S10 ), and at least 75.3% of the gained genes showed evidence of transcription. Some of the gained genes were obtained by gene duplication. For example, we detected five copies of FBXO31 based on synteny analysis, whereas an additional 52 FBXO31 genes could be identified in the M. brandtii genome. This protein mediates DNA damage-induced growth arrest by targeting CDK1 for ubiquitin-mediated degradation. Several studies have reported a relatively recent wave of DNA transposon activity in M. lucifugus (but not megabats or other mammals), which may have contributed to the M. brandtii gene duplication [12] . We also identified 194 pseudogenes, containing 142 frameshift and 72 premature termination events ( Supplementary Data 3 ). A salient example is the gulonolactone ( L -) oxidase ( GULOP ) gene. As is the case for primates, the ability to synthesize vitamin C is lost in bats [13] . In agreement with this observation and a recent study that examined the related M. lucifugus [14] , we found that this gene is inactivated in M. brandtii ( Supplementary Fig. S8 ). Echolocation Amino-acid residues that are uniquely altered in the bat lineage alone or in bats and species with similar phenotypes, such as powered flight in bats and birds and echolocation in bats and dolphins, can reveal clues about functional adaptations. We examined amino-acid changes at evolutionary conserved residues of orthologs in 48 vertebrate genomes ( Supplementary Table S11 ) and identified four proteins with unique amino-acid changes that are common to the echolocating mammals the Brandt’s bat and the Atlantic bottlenose dolphin, Tursiops truncatus ( Table 2 ). Interestingly, two of these genes ( SLC45A2 and RGS7BP ) are expressed in the inner ear. SLC45A2 ( Supplementary Fig. S9 ) is a transporter protein that has an important role in melanin synthesis [15] and was recently reported to be one of the most abundantly expressed genes in the inner ear [16] . Melanin is highly sound-absorbing [17] and may function in the inner ear to protect the cochlea from aging-related hearing loss and sound stressors in much the same manner as melanin in the skin protects against ultraviolet light [18] , [19] , [20] . A recent study found that RGS7BP ( Supplementary Fig. S10 ) is expressed in vestibular ganglion neurons in the inner ear, which are important for spatial orientation [21] . These findings add to the list of independent gene loci with putative functions in the inner ear of echolocating bats and dolphins, such as prestin (also known as SLC26A5) [22] , TMC1 [23] , DFNB59 [23] , SLC45A2 and RGS7BP , implicating them in echolocation. Table 2 Proteins with unique residues in Myotis and dolphin. Full size table Among the positively selected genes in the Brandt’s bat, we found additional genes with potential roles in echolocation ( Supplementary Table S12 ): TRPV5 (TRPC channels have a role in mechanosensation, including hearing and proprioception) and NOX3 (highly expressed in the inner ear and involved in the biogenesis of otoconia/otolith—the crystalline structures for perception of gravity). GO categories significantly enriched (Benjamini–Hochberg false discovery rate (FDR) adjusted P -value <0.05) in the set with evidence for positive selection in the Brandt’s bat included genes associated with immunity and fertilization ( Supplementary Table S13 ). Our analysis also revealed that 21 M. brandtii genes contained at least one unique amino-acid change ( Supplementary Table S14 ). Notable among them were genes associated with visual function ( CNGB3 ), reproduction ( FSHB , DDX4 , HARS2 , PRSS23 and PHTF1 ), Wnt signalling ( APC ), RNA interference ( ERI3 ) and helicase activity ( DDX1 , DDX4 , HELB and VPS4B ). Vision The small eyes of echolocating bats are adapted for use beyond the range of echolocation [24] , as well as for short-range navigation in concert with echolocation [25] . Molecular innovation of photopigment opsins, rhodopsin and downstream signalling components may, therefore, confer an advantage to echolocating bats at dawn and dusk ( Supplementary Note 2 ). Indeed, we found changes in photoreceptor genes of the Brandt’s bat suggestive of adaptation to dim-light conditions ( Supplementary Fig. S11 ) and UV vision ( Supplementary Fig. S12 ). CNGB3 (cyclic nucleotide gated channel beta 3) codes for one of the two proteins necessary for sensory transduction of cone photoreceptors. Mutations in this gene result in impaired conversion of light captured by cone opsins to nerve impulses and CNGB3 mutations have been associated with achromatopsia [26] , [27] , where subjects can only see clearly at low light levels. Although their cone photoreceptor cells remain structurally intact, signalling is blunted and they are either totally or partially colour blind and display reduced visual capacity in bright light (day-blindness). M. brandtii , M. lucifugus and E. fuscus , which roost in caves during the day, harbour a unique amino-acid change in the transmembrane domain S5 of CNGB3 ( Supplementary Fig. S13 ), where a tyrosine highly conserved in vertebrates is replaced with cysteine. Interestingly, M. lucifugus avoids obstacles better under dim-light conditions such as dusk than under bright daylight [25] , [28] . We hypothesize that the CNGB3 amino-acid change is a loss-of-function mutation that result in day-blindness in strictly nocturnal, echolocating bats. It will be of future interest to obtain the genome or retinal transcriptome data from additional bat species. Hibernation and reproduction Hibernation is a hypometabolic state in mammals wherein they enter a state of torpor, typically in response to environmental conditions such as a lack of food (insects in the case of M. brandtii ) and subzero temperatures [29] . To obtain insights into this adaptation, we examined gene expression in the liver of M. brandtii subjected to hibernation for 6 months ( Supplementary Table S15 and Supplementary Data 4 ). 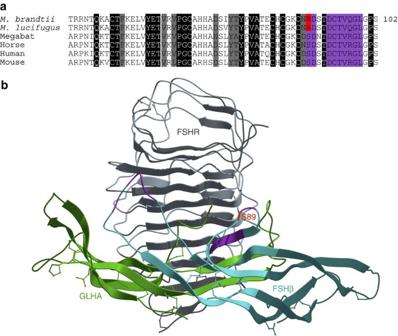Figure 3: FSHβ of the Brandt’s bat harbours a radical amino-acid substitution in a conserved position. (a) Alignment ofFSHB-encoded peptide sequences. Amino-acid numbering corresponds to the mature FSHβ peptide. (b) Structural model of FSHβ (cyan), the follicle-stimulating hormone receptor FSHR (grey) and the glycoprotein hormones α chain GLHA/FSHα (green) (PDB ID code 1xwd). In both subfigures, FSHβ residues buried at the FSHR receptor–ligand interface are highlighted in purple, while a radical amino-acid substitution within the interface in bats with delayed ovulation is shown in red. This analysis revealed an enrichment (Benjamini–Hochberg FDR-adjusted P -value <0.05) of downregulated genes associated with RNA binding (GO:0003723) and structural integrity of the ribosome (GO:0003735) ( Table 3 ). In addition, downregulated genes have roles in protein synthesis (multiple ribosomal proteins, NACA , and PRPS1 ; GO:0003723), as well as glycolysis ( ENO1 and GAPDH ), splicing ( SNRPC ) and mitochondrial respiration ( NDUFA3 ). Enriched gene categories upregulated during hibernation included digestion (metabolism; GO:0007586) and peptidase activity ( Table 3 ). We also observed genes involved in lipid metabolism ( PLA2G1B , CEL , UNQ599 , G0S2 , CYP4X1 and CLPS ), coagulation ( CPB1 and MBL1 ), maintenance of oxidative stress ( OSGIN1 and LYPD3 ) and adaptation to starvation ( FGF21 and ATG101 ). Overall, these changes are consistent with the expected [29] shift from carbohydrate to lipid metabolism and the reduction in protein synthesis during the hypometabolic state of hibernation. Table 3 Significant GO categories of hibernating M. brandtii . Full size table In Myotis , mating occurs right before or during hibernation, where males can mate with torpid females. The sperm is then stored in the female reproductive tract, with ovulation and fertilization delayed until spring [30] . Follicle-stimulating hormone (FSH) is a glycoprotein hormone consisting of a common α-subunit and a hormone-specific β-subunit. The hormone binds to its cognate G-protein-coupled receptor (FSH receptor; FSHR) in the testis and ovary and, together with luteinizing hormone (LH) and its receptor (LHR), is produced in the anterior pituitary and essential for reproduction. We found a unique amino-acid change (S89R) of potential functional significance in the mature FSH beta-subunit (FSHβ) peptide of hibernating bats ( Fig. 3 and Supplementary Fig. S14 ). This change occurs within the hydrophobic receptor–ligand interface that determines receptor-binding specificity [31] , and the replacement of a small amino acid with a large, charged one would be expected to disrupt the FSHβ–FSHR interaction. Interestingly, it has recently been hypothesized [31] that Ser89 may explain why LH cannot bind FSHR. LH, encoded by LHB , is a paralogous gene to FSHB and the LH beta-subunit (LHβ) is similar to FSHβ but harbours arginine at the site homologous to Ser89. Moreover, site-directed mutagenesis of residues 88–91 of FSHβ (DSDS) to the LHβ sequence (RRST) allows FSHβ to bind LHR [32] . A study of the Asiatic greater yellow house bat ( Scotophilus heathi ), which is in the same family as M. brandtii, suggests that increased responsiveness to LH could be associated with delayed ovulation [33] . Taken together, we hypothesize that an aberrant gonadotropin system, where FSH may have reduced affinity for FSHR and a gain-of-affinity for LHR, may contribute to the delayed ovulation observed in many bat species. Future studies using, for example, knock-in mice expressing a Ser89Arg mutation, should provide interesting insights into the phenotypic consequences of this amino-acid change. Figure 3: FSHβ of the Brandt’s bat harbours a radical amino-acid substitution in a conserved position. ( a ) Alignment of FSHB -encoded peptide sequences. Amino-acid numbering corresponds to the mature FSHβ peptide. ( b ) Structural model of FSHβ (cyan), the follicle-stimulating hormone receptor FSHR (grey) and the glycoprotein hormones α chain GLHA/FSHα (green) (PDB ID code 1xwd). In both subfigures, FSHβ residues buried at the FSHR receptor–ligand interface are highlighted in purple, while a radical amino-acid substitution within the interface in bats with delayed ovulation is shown in red. Full size image Potential adaptations for extended lifespan in bats Growth hormone (GH) insensitivity encompasses a range of genetic abnormalities of the GH/IGF1 axis. Mutations in the single-transmembrane receptor GHR, including the transmembrane domain-coding exon 8, have been shown to result in human Laron-type dwarfism (short-stature), a subtype of GH insensitivity [34] . Interestingly, GHR mutations or GHR dysfunctions have been associated with increased resistance to diabetes and cancer in humans and mice [35] , [36] , [37] . We found that Leu284 in the transmembrane domain of GHR, which is highly conserved in tetrapods, is deleted in M. brandtii , M. lucifugus and two other echolocating bat species, the big brown bat ( Eptesicus fuscus ) and the Mexican free-tailed bat ( Tadarida brasiliensis ) ( Fig. 4a and Supplementary Fig. S15 ). In contrast, the echolocating Jamaican fruit bat ( Artibeus jamaicenis ) and the megabat ( Pteropus vampyrus ) do not harbour this deletion. In addition, the nearby Ile275 is uniquely replaced with methionine in M. brandtii , M. lucifugus , E. fuscus and T. brasiliensis . GH binding induces conformational changes thought to be mediated by the GHR transmembrane domain [38] . Furthermore, mutations in the transmembrane domain of closely related receptors have been observed to alter their function [39] . The GHR transmembrane residue deletion is present in the Vespertilionoidea superfamily, which comprises the largest number of species in the Chiroptera suborder Yangochiroptera. This superfamily includes the Vespertilionidae family, commonly known as Vesper bats (the 4–8 g M. brandtii , the 6.8 g M. lucifugus , the 16.9 g E. fuscus ) [40] and the Molossidae family (the 11.2 g T. brasiliensis) [40] . The GHR transmembrane residue deletion is not present in the Jamaican fruit bat (the 39.8 g A. jamaicenis [40] ) in the family Phyllostomidae. These data suggest that the amino-acid deletion appeared after the divergence between Vespertilionoidea and the branch leading to New World leaf-nosed bats (Phyllostomidae) ~50 million years ago [41] . 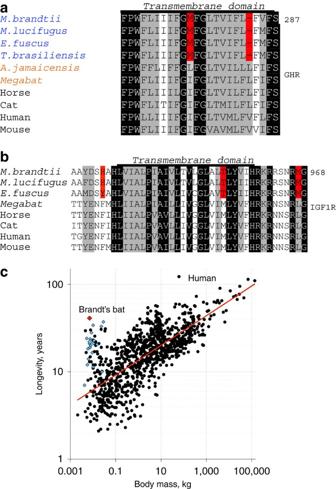Figure 4: Adaptations in the GH/IGF1 axis of the Brandt’s bat and its much longer lifespan than expected for its body size. (a) Alignment of mammalian GHR protein sequences. An amino-acid deletion at position 284 and a methionine at position 275 unique to bats in the Vespertilionoidea superfamily are shown in red. Insect-eating bats are shown in blue and fruit-eating bats in orange. (b) Alignment of mammalian IGF1R protein sequences. Unique amino-acid replacements in bats in the Vespertilionoidea superfamily are highlighted in red. Identical residues and similar residues are shaded in black and grey, respectively. (c) Correlation between body mass and maximum lifespan in mammals.Myotisbats are shown as blue diamonds, and other mammals as grey circles. The Brandt’s bat is indicated by a red diamond. Figure 4: Adaptations in the GH/IGF1 axis of the Brandt’s bat and its much longer lifespan than expected for its body size. ( a ) Alignment of mammalian GHR protein sequences. An amino-acid deletion at position 284 and a methionine at position 275 unique to bats in the Vespertilionoidea superfamily are shown in red. Insect-eating bats are shown in blue and fruit-eating bats in orange. ( b ) Alignment of mammalian IGF1R protein sequences. Unique amino-acid replacements in bats in the Vespertilionoidea superfamily are highlighted in red. Identical residues and similar residues are shaded in black and grey, respectively. ( c ) Correlation between body mass and maximum lifespan in mammals. Myotis bats are shown as blue diamonds, and other mammals as grey circles. The Brandt’s bat is indicated by a red diamond. Full size image We also found changes in the M. brandtii IGF1R sequence, another key aging-related gene that is tightly intertwined with GHR function. Experiments in Caenorhabditis elegans found that knockout of daf-2 , a functional homologue of IGF1R and the insulin receptor, extends lifespan several-fold [42] . The single-transmembrane domain (amino acids 936–959) of IGF1R is highly conserved in mammals, including the megabat, but in M. brandtii , M. lucifugus and E. fuscus we observed multiple unique changes both in the transmembrane region (M954T) and immediately preceding (F933H) and following (L967M) it ( Fig. 4b and Supplementary Fig. S16 ). The transmembrane region could not be retrieved from transcriptomic data of T. brasiliensis and A. jamaicenis . This domain is important for signal transduction in response to binding of IGF1, and both mutations within this region and deletion of amino acids immediately preceding it affect IGF1R function [43] . To gain further insights into the evolved GH/IGF1 axis, we compared gene expression between mouse and Brandt’s bat livers ( Supplementary Note 3 ). If M. brandtii GHR is dysfunctional and bats display a phenotype corresponding to that of long-lived GHR −/− mice, one would expect insulin signalling in the liver of the Brandt’s bat similar to the changes observed in the GHR −/− mouse liver [44] . Several insulin signalling-associated genes, including the major mediator of insulin action, forkhead box protein O1 ( FOXO1 ), were expressed at a higher level in both M. brandtii and GHR −/− mice compared with wild-type mice ( Supplementary Table S16 ). Dysregulated expression of insulin homeostasis genes in the liver of GHR −/− mice is caused by the ablation of GH signalling in these animals. GHR −/− mice exhibit an altered pancreatic structure, with small islets of Langerhans and decreased β-cell mass [45] . We examined the pancreas of M. brandtii ( Supplementary Note 4 ) and observed a similar phenotype ( Supplementary Fig. S17 ). We further compared M. brandtii gene expression to those of several long-lived mice [46] ( Supplementary Note 5 ). M. brandtii exhibited the same gene expression changes for 11 out of 15 orthologous genes differentially expressed in long-lived mice compared with wild-type strains ( Supplementary Table S17 ). Finally, we assembled the mitochondrial genome of M. brandtii ( Supplementary Fig. S18 ) and analysed the amino-acid content of its genes. It has been hypothesized that a relationship exists between reduced number of cysteine in mitochondrially encoded proteins and longevity [47] , [48] . We found that cysteine content of mitochondria-encoded proteins was much lower than that expected based on its body mass and slightly higher than expected based on lifespan ( Supplementary Fig. S19 ). In this regard, the Brandt’s bat is more similar to large-sized animals ( Fig. 4c and Supplementary Fig. S19 ). However, additional factors (such as phylogenetic bias) may influence this correlation [49] , [50] . The Brandt’s bat possesses features attributed to increased longevity of bats [40] : it hibernates, has a low reproductive rate and roosts in caves (thus, avoiding predators and extreme weather conditions). Like larger mammals, this bat exhibits long reproductive cycles, long time to maturity and a long lifespan. The Brandt’s bat produces a single pup, which may account for 10–15% of the adult body mass. It is prudent to ask whether the changes in the GHR/IGF1 axis in the Brand’s bat contribute to the animal’s long lifespan, its small body size or both. The prevailing evidence is that early mammals, including the earliest horses, had a small body size [51] , [52] . Although the body size of most mammals and their extinct relatives has since increased, the body size of bats is much more diverse. Recent work supports the hypothesis that the body size of bats correlates with the echolocation and flight traits as well as dietary specializations, where a small body size is advantageous for echolocating animals that feed on small, fast-moving insects [53] . In contrast, a larger body size may be advantageous for bat species, some of which do not echolocate, that feed on bigger, slow-moving insects or fish or fruits. Echolocating insectivorous bats smaller than the Brandt’s bat, such as the distantly related 2 g bumblebee bat Craseonycteris thonglongyai in the suborder Yinpterochiroptera [54] , but with unknown maximum lifespans, exist. Although it is appreciated that other genes have been altered during the ~82 million years of bat evolution, we suggest that the changes observed in GHR and IGF1R contribute to the longevity and dwarfism-like phenotype of the Brandt’s bat. Moreover, M. brandtii may mirror GHR dysfunction in mice and humans, and possibly insulin signalling in long-lived nematodes. Taken together, we suggest that the combination of adaptations, such as hibernation, low reproductive rate, cave roosting and an altered GH/IGF1 axis, serve to extend the Brandt’s bat lifespan. Our observations are pertinent to the Yangochiroptera suborder of echolocating bats, the second and most numerous suborder of bats (Chiroptera). It will be important for future studies to compare these findings to long-lived, small, echolocating bats of the suborder Yinpterochiroptera (which includes the non-echolocating megabat, P. vampyrus , examined in this study). Further analyses, including sequencing and lifespan studies (such as banding schemes) are required to fully determine the role of the GHR/IGF1 axis in the longevity and body size of bats. Following submission of our Brandt’s bat genome study, an article on the genomes of the related David’s Myotis ( Myotis davidii ) and the megabat the black flying fox ( Pteropus alecto ) was published [55] . Although the other study examined different aspects of bat biology, the availability of two additional bat genomes should greatly help in further analyses of longevity and other traits reported in our study. In summary, genome and transcriptome analyses of a mammal with a most exceptional lifespan provide clues to its evolution and several unique traits. The generated data sets can be further mined and the identified genes characterized, helping to explain the basis for powered flight, echolocation, hibernation, small body size and most importantly, the basis for the remarkable longevity of this animal, and bats in general. Animal sampling Male M. brandtii bats were collected at a hibernation roost in the Perm Krai, Russia (GPS coordinates N 58 50.089 E 57 36.716) in December 2011 and April 2012, and at a summer roost in Kirov Oblast, Russia (GPS coordinates N 57 25.000 E 48 54.500) in June 2012 ( Fig. 1 ). Animals were killed on-site and tissues frozen in liquid nitrogen. The sequenced individual bat was a hibernating adult male from the Obvalnaya cave in the Perm Krai. Liver, kidney and brain transcriptomes were from both hibernating and summer-active adult males. All procedures were carried out in accordance with guidelines of the Animal Ethics Committee of the Russian Academy of Sciences. Genome sequencing and annotation The M. brandtii genome and transcriptomes were sequenced on the Illumina HiSeq 2000 platform. The genome was assembled using the de Bruijn graph-based assembler SOAP denovo [56] . Full description and associated references for sequencing, assembly and gene annotation are provided as Supplementary Methods . Identification of proteins with unique amino-acid changes An in-house Perl pipeline was used to identify orthologous protein sites where types/groups of residues are shared by Brandt’s and other species of interest. In addition to the Brandt’s bat, 47 vertebrate species were examined. Briefly, two Perl scripts were employed: the first script identified amino-acid residues conserved in all sequences except the species of interest (for example, a valine in M. brandtii , and an alanine in all other organisms). As genome-wide comparisons of radical amino-acid changes may be more likely to reflect functional diversification, a second Perl script was employed to scan orthologous protein sites where types/groups of residues were shared by Myotis alone or with other species of interest. It is generally assumed that radical amino-acid changes are much more likely to reflect functional diversification, and the second script revealed if M. brandtii and M. lucifugus (plus other species of interest) harbour residue changes in four groups of amino acids: acidic (ED), basic (KHR), cysteine (C) and ‘other’ (STYNQGAVLIFPMW). For example, two species harbour K and H, although the other organisms contain either acidic, cysteine or ‘other’ residues at a particular site. Candidates were manually examined for alignment quality and conservation of the region with amino-acid changes. Raw M. brandtii genome and transcriptome data were examined to further exclude gene misprediction and misannotations. See Supplementary Methods for further details. Identification of genes under positive selection To detect positive selection, we examined 1:1 orthologous protein-coding sequence alignments of Brandt’s bat, the megabat P. vampyrus , dog, horse, cow and the dolphin Tursiops truncatus . Briefly, the strict branch-site model in the CodeML program of the PAML (phylogenetic analysis using maximum likelihood) package (v4.6; settings: model=2, NS sites=2) [57] was employed. The branch-site test for positive selection assumes that the branches in the phylogenetic tree can be divided into foreground branches (where codons are under positive selection) and background branches (where positive selection is absent) [57] . Model A1 (H 0 ; CodeML settings: fix_omega=1, omega=1), where a codon may evolve neutrally or under purifying selection was compared with model A, where codons on the branch of interest can be under positive selection (H A ; CodeML settings: fix_omega=0, omega=1). Likelihood ratio test P -values were computed assuming that the null distribution was a χ 2 -distribution with 1 degree of freedom and adjusted for multiple testing with a FDR threshold of 0.05. If significant, codon sites with a Bayes empirical Bayes probability >95% were considered to be under positive selection. We manually examined a subset of PAML results significant at a 1% FDR. Large, divergent protein families and proteins with coiled-coil domains were omitted from the analysis. See Supplementary Methods for greater detail. Transcriptome sequencing and analyses Total RNA was isolated from livers, kidneys and brains of animals sampled in December 2011 (hibernated for 2 months), April 2012 (hibernated for 6 months) and June 2012 (summer-active animals). RNA sequencing libraries were constructed using the Illumina mRNA-Seq Prep Kit. Briefly, oligo(dT) magnetic beads were used to purify mRNA molecules. The mRNA was further fragmented and randomly primed during the first-strand synthesis by reverse transcription. This procedure was followed by second-strand synthesis with DNA polymerase I to create double-stranded cDNA fragments. The double-stranded cDNA was subjected to end repair by Klenow and T4 DNA polymerases and A-tailed by Klenow lacking exonuclease activity. Ligation to Illumina Paired-End Sequencing adapters, size selection by gel electrophoresis and PCR amplification completed the library preparation. The 200 bp paired-end libraries were sequenced using Illumina HiSeq 2000 (90 bp at each end). Transcriptome reads were mapped by TopHat [58] , and mapped reads were analysed with in-house Perl scripts. Differentially expressed genes were calculated using the GFOLD package [59] . Briefly, GFOLD (generalized fold change) assigns reliable statistics for expression changes based on the posterior distribution of log fold change. Read counts were obtained from TopHat-generated BAM files using SAMtools [60] and differentially expressed genes identified by comparing the gene expression in the liver of hibernating and summer-active bats, exactly as outlined in the GFOLD manual. Accession codes : The Brandt’s bat whole-genome shotgun project has been deposited at GenBank under the accession code ANKR00000000 . The version described in this paper is the first version, ANKR01000000. All short read data have been deposited into the Short Read Archive under the accession code SRA061140 . Raw sequencing data of the transcriptome have been deposited in Gene Expression Omnibus (GEO) with the accession code GSE42297 . How to cite this article: Seim, I. et al . Genome analysis reveals insights into physiology and longevity of the Brandt’s bat Myotis brandtii. Nat. Commun. 4:2212 doi: 10.1038/ncomms3212 (2013)